Retinoid-independent motor neurogenesis from human embryonic stem cells reveals a medial columnar ground state A major challenge in neurobiology is to understand mechanisms underlying human neuronal diversification. Motor neurons (MNs) represent a diverse collection of neuronal subtypes, displaying differential vulnerability in different human neurodegenerative diseases. The ability to manipulate cell subtype diversification is critical to establish accurate, clinically relevant in vitro disease models. Retinoid signalling contributes to caudal precursor specification and subsequent MN subtype diversification. Here we investigate the necessity for retinoic acid in motor neurogenesis from human embryonic stem cells. We show that activin/nodal signalling inhibition, followed by sonic hedgehog agonist treatment, is sufficient for MN precursor specification, which occurs even in the presence of retinoid pathway antagonists. Importantly, precursors mature into HB9/ChAT-expressing functional MNs. Furthermore, retinoid-independent motor neurogenesis results in a ground state biased to caudal, medial motor columnar identities from which a greater retinoid-dependent diversity of MNs, including those of lateral motor columns, can be selectively derived in vitro . The ability to generate defined neuronal lineages from human embryonic stem cells (hESCs) through application of developmental principles offers an unprecedented opportunity to interrogate the molecular mechanism(s) underlying human neuronal diversity [1] , [2] . Although often considered a single group, spinal motor neurons (MNs) are a collection of diverse neuronal subtypes that in turn have distinct connectivity and also display differential vulnerability in diseases such as amyotrophic lateral sclerosis and spinal muscular atrophy [3] . This highlights the need for subtype-specific MN differentiation protocols, which will in turn permit more accurate and clinically relevant in vitro model systems of motor neuronopathies. Insights from spinal cord neuronal fate specification have greatly informed our understanding of the generation of neuronal diversity and highlight common themes underlying neuronal identity and organization based on signalling along the rostrocaudal (R-C) and dorsoventral (D-V) axes [4] , [5] . Default models of neurogenesis commonly suggest an initial rostral positional identity of resulting precursors [6] , [7] . Progressive re-specification of rostral to more caudal fates is choreographed by a number of signalling pathways, including fibroblast growth factors (FGFs) [8] , retinoic acid (RA) [9] , transforming growth factor-β (TGF-β) [10] and WNTs [11] . R-C patterning of the caudal hindbrain and rostral spinal cord are regulated through graded RA signalling, in concert with WNTs and FGFs, and establish positional boundaries of HOX gene expression. Significantly, the absence of RA signalling results in specific abnormalities in R-C and also in D-V organization [12] . Once caudalized, ventral neuronal fate specification is initiated by sonic hedgehog (SHH) signalling through its effects on both homeodomain (HD) and basic helix-loop-helix transcription factors, and is believed to occur via a de-repression strategy [13] . Within the D-V axis, SHH promotes the expression of class II transcription factors (OLIG2, NKX2.2 and NKX6.1), whereas RA promotes the expression of class 1 factors (PAX7, PAX6 and IRX3). HD and basic helix-loop-helix transcription factors across both classes function in combination to establish discrete precursor domains [5] . MN precursors arising from the pMN domain are defined by expression of the transcription factors NKX6.1, OLIG2 and NEUROG2 [14] , [15] , [16] . Their combined action directs MN precursors to a post-mitotic state, after which they upregulate fate consolidating genes such as HB9 [17] , [18] . Beyond precursor specification, retinoid signalling is required to diversify MN subtypes from the common MN precursor pool and establish spinal cord columnar organization. Spinal motor column precursor cells are partitioned to lateral and medial pools, acquire different fates with respect to axonal trajection and target innervation and can be discriminated based on their gene expression profiles [19] , [20] . RA is required for development of somatic MNs in the caudal hindbrain [21] and lateral motor column (LMC) MNs. Within the LMCs at brachio-lumbar foci, RA is synthesized locally by subpopulations of MNs (expressing RALDH2) and regulates the differentiation of migrating neurons into subsets of LMC neurons. Ectopic RA synthesis affects MN subtype specification [22] and ectopic RALDH2 expression in spinal neurons generates LMC MNs, while RALDH2 knockdown and knockouts cause a reduction, but not complete elimination, of both lateral and medial LMC neurons [20] , [23] . Together, these studies highlight distinct requirements for RA signalling in MN generation and organization. Application of developmental inductive signals, such as RA and SHH, has enabled directed differentiation of MNs from mouse and human ESCs [1] , [24] . Inhibition of activin/nodal signalling accelerates neural conversion from hESCs [25] and additionally imposes a caudal positional identity on resulting precursors [26] . This allows study of the requirement for RA in spinal motor neurogenesis beyond its ability to induce caudal fate specification. We therefore addressed whether human motor neurogenesis can be achieved independently of retinoid signalling using small molecule-directed differentiation of hESC fate.In this study, we show the accelerated generation of predominantly caudal functional MNs that is independent of retinoid signalling. Importantly, retinoid-independent differentiation reveals a novel approach to MN generation and their subtype diversification in vitro . SB431542 accelerates MN precursor specification from hESCs We previously demonstrated that the activin/nodal receptor kinase (ALK4/5/7) inhibitor SB431542 accelerates efficient conversion of hESCs to predominantly caudal neural precursors [26] . To investigate whether accelerated MN precursor specification could be achieved in these cultures, we applied a standard programme of morphogenetic cues [1] . Day 4 SB431542-treated cells were exposed to FGF2, RA and the SHH agonist puromorphamine for 8 days. The resulting aggregates demonstrated significant upregulation of the MN lineage transcription factors OLIG2 and ISLET1 ( Fig. 1a–i ), which on terminal differentiation generated mature SYNAPSIN-positive neurons, with 17.5±1.2% of cells co-expressing HB9/β-III-TUBULIN, confirming MN identity ( Fig. 1j–l ). 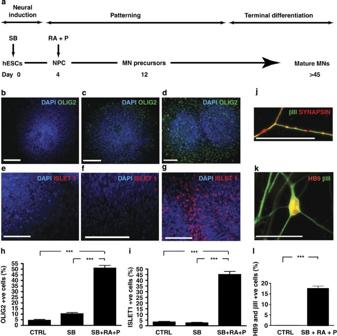Figure 1: Accelerated motor neurogenesis from human embryonic stem cells. (a) The small compound SB431542 (an inhibitor of the activin/nodal signalling pathway) was used for neural conversion of human embryonic stem cells (hESCs). SB431542 was added at day 0 followed by retinoic acid and a sonic hedgehog agonist called puromorphamine. OLIG2 immunocytochemistry (green) of day 12 hESC-NPCs neuralized in (b) chemically defined medium alone, (c) 10 μM SB431542 from days 0 to 4 or (d) SB431542 exposure from days 0 to 4, followed by 0.1 μM retinoic acid and 1 μM puromorphamine for a further 8 days. ISLET1 immunocytochemistry (red) of day 12 hESCs neuralized in (e) chemically defined medium alone, (f) 10 μM SB431542 from days 0 to 4, (g) SB431542 exposure from days 0 to 4, followed by 0.1 μM retinoic acid and 1 μM puromorphamine for a further 8 days. All cultures were treated with 10 ng ml−1FGF2 from days 4 to 12. Quantitative immunocytochemical analysis of (h) OLIG2 and (i) ISLET1 is shown. Following the protocol detailed inaand in the continued presence of retinoic acid, cells were plated down for terminal differentiation. (j) β-III-TUBULIN/SYNAPSIN expression occurs within 4–7 days, and (k) HB9 expression within neuronal nuclei occurs after 4–5 weeks of terminal differentiation. (l) Quantitative immunocytochemistry for HB9/β-III-TUBULIN (βIII) co-expressing cells. Error bars inh–jrepresent s.e.m, ***P<0.001, Mann–Whitney rank-sum test, a minimum of three biological repeats were performed for each experiment. DAPI, 4,6-diamidino-2-phenylindole; hESC, human embryonic stem cell; MN, motor neuron; NPC, neural precursor cell; P, puromorphamine (a sonic hedgehog agonist); RA, retinoic acid; and SB, SB431542 (an inhibitor of the activin/nodal signalling pathway). Scale bars (b–g) 100 μm; (j,k) 25 μm. Figure 1: Accelerated motor neurogenesis from human embryonic stem cells. ( a ) The small compound SB431542 (an inhibitor of the activin/nodal signalling pathway) was used for neural conversion of human embryonic stem cells (hESCs). SB431542 was added at day 0 followed by retinoic acid and a sonic hedgehog agonist called puromorphamine. OLIG2 immunocytochemistry (green) of day 12 hESC-NPCs neuralized in ( b ) chemically defined medium alone, ( c ) 10 μM SB431542 from days 0 to 4 or ( d ) SB431542 exposure from days 0 to 4, followed by 0.1 μM retinoic acid and 1 μM puromorphamine for a further 8 days. ISLET1 immunocytochemistry (red) of day 12 hESCs neuralized in ( e ) chemically defined medium alone, ( f ) 10 μM SB431542 from days 0 to 4, ( g ) SB431542 exposure from days 0 to 4, followed by 0.1 μM retinoic acid and 1 μM puromorphamine for a further 8 days. All cultures were treated with 10 ng ml −1 FGF2 from days 4 to 12. Quantitative immunocytochemical analysis of ( h ) OLIG2 and ( i ) ISLET1 is shown. Following the protocol detailed in a and in the continued presence of retinoic acid, cells were plated down for terminal differentiation. ( j ) β-III-TUBULIN/SYNAPSIN expression occurs within 4–7 days, and ( k ) HB9 expression within neuronal nuclei occurs after 4–5 weeks of terminal differentiation. ( l ) Quantitative immunocytochemistry for HB9/β-III-TUBULIN (βIII) co-expressing cells. Error bars in h–j represent s.e.m, *** P <0.001, Mann–Whitney rank-sum test, a minimum of three biological repeats were performed for each experiment. DAPI, 4,6-diamidino-2-phenylindole; hESC, human embryonic stem cell; MN, motor neuron; NPC, neural precursor cell; P, puromorphamine (a sonic hedgehog agonist); RA, retinoic acid; and SB, SB431542 (an inhibitor of the activin/nodal signalling pathway). Scale bars ( b–g ) 100 μm; ( j , k ) 25 μm. Full size image MN induction can occur independently of retinoid signalling The imposition of caudal positional identity by SB431542, demonstrated by the upregulation of HOX genes and downregulation of anterior markers OTX2 and PAX6, has previously been reported [26] . Importantly, the upregulation of HOX genes in SB431542-treated cultures occurs independently of exogenous RA. As a primary function of RA in MN specification from ESCs is to induce HOX gene expression [27] , we reasoned that MN specification might be achieved independently of exogenous RA in SB431542-neuralized hESC cultures. Addition of puromorphamine to SB431542-treated cultures resulted in significant upregulation of OLIG2, independently of exogenous RA ( Fig. 2a–d ). Furthermore, SYNAPSIN/β-III-TUBULIN co-immunolabelling and HB9/β-III-TUBULIN quantitative immunocytochemistry confirmed the presence of mature MNs ( Fig. 2e–g , 11.2±0.9%). To further confirm retinoid-independent MN specification, we next differentiated hESCs in the presence of the RAR and RXR retinoid receptor antagonists UVI2024 and UVI3003 (refs 28 , 29 ). The efficacy of these compounds was confirmed by demonstrating inhibition of RA-induced HOXB4 and HOXC5 gene expression in control cultures ( Supplementary Fig. S1 ). In cultures treated with puromorphamine in the continued presence of UVI2024 and UVI3003 and without exogenous RA, OLIG2 was still significantly upregulated ( Fig. 2a–d ). There was no statistically significant difference in the number of OLIG2-expressing cells when comparing both retinoid-free culture methods ( Fig. 2d ), suggesting a phenotypically inconsequential level of endogenous retinoid signalling. Crucially, terminal differentiation of the resulting precursors in the continued presence of UVI2024 and UVI3003 generated neurons expressing classical MN markers, including NGN2, ISL1, ChAT and VAChT, detected by reverse transcription PCR (RT–PCR) as well as positive immunocytochemistry for MN lineage markers NKX6.1, ISL1, HB9, ChAT, SMI32 and LHX3 ( Supplementary Fig. S2 ). Furthermore, SYNAPSIN/β-III-TUBULIN co-immunolabelling and HB9/β-III-TUBULIN quantitative immunocytochemistry confirmed the presence of mature MNs ( Fig. 2e–g , 12.0±1.3%). In addition to MNs, retinoid-independent cultures most likely contain ventral interneuronal subtypes. This was investigated by LHX3/β-III-TUBULIN quantitative immunocytochemistry ( Supplementary Fig. S2 ). Given that the cultures were comprised of 29.4±1.3% LHX3+/β-III-TUBULIN+ cells and 9.7±0.8% total MNs at 9 weeks post mitogen withdrawal, a portion of the cultures were likely to be V2 interneurons, consistent with previous reports [1] , [24] . 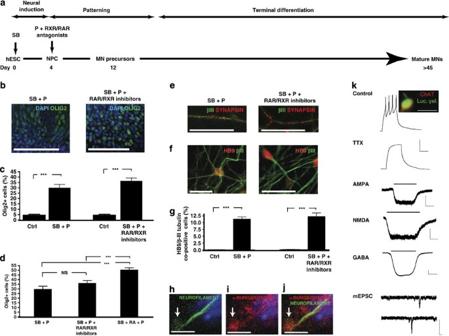Figure 2: Retinoid-independent motor neurogenesis from human embryonic stem cells. (a) SB431542 treatment from day 0 to 4 followed by puromorphamine from day 4 to 12, with pan-retinoid antagonists from day 4 onwards. (b) OLIG2 immunocytochemistry (green) of day 12 hESC-NPCs derived in retinoid-free conditions (−/+ pan-retinoid antagonists). Quantitative OLIG2 immunocytochemistry comparing retinoid-independent culture conditions with (c) control conditions and (d) retinoid-treated conditions. All cultures were treated with 10 ng ml−1FGF2 from day 4 to 12. On terminal differentiation (e) β-III-TUBULIN (βIII)/SYNAPSIN expression occurs within 4–7 days and (f) HB9 expression after 4–5 weeks. (g) Quantitative immunocytochemistry for HB9/β-III-TUBULIN co-expressing cells. Co-culture of RA-independent MN precursors with C2C12-derived myotubes for 12 days results in (h) outgrowth of neurite tips, (i) Tetramethyl Rhodamine Iso-Thiocyanate (TRITC)-α-bungarotoxin plaques on myotubes and (j) neuromuscular synapse formation. (k) Current-clamp recording from RA-independent MNs (56 days post-plating): injection of positive current generates action potentials that are blocked by voltage-dependent Na+channel blocker tetrodotoxin (TTX; 300 nM). Voltage-clamp recordings from RA-independent MNs, held at −60 mV, showing responses to application of the ionotropic glutamate receptor agonists α-amino-3-hydroxyl-5-methyl-4-isoxazole-propionate (AMPA; 50 μM) andN-methyl-D-aspartic acid (NMDA; 100 μM) and to the inhibitory neurotransmitter, γ-aminobutyric acid (GABA; 50 μM). The lower two traces in this panel show TTX-insensitive miniature excitatory postsynaptic currents (mESPCs), recorded in the presence of picrotoxin (50 μM) and under conditions in which NMDA receptors would be blocked by magnesium ions (Mg2+) present in the external recording solution. Calibration bars for current-clamp recordings, 16 mV and 400 ms; for agonist-evoked whole-cell currents, 80 pA and 4 s; and for mEPSCs, 16 pA and 80 ms. To confirm MN identity,post hocstaining with choline acetyltransferase (ChAT) was conducted. Error bars inc,dandgrepresent s.e.m, ***P<0.001, Mann–Whitney rank-sum test, a minimum of three biological repeats were performed for each experiment. Ctrl, control; DAPI, 4,6-diamidino-2-phenylindole; mESPCs, miniature excitatory postsynaptic currents; MN, motor neuron; NS, not significant; NPC, neural precursor cell; P, puromorphamine (sonic hedgehog agonist); RA, retinoic acid; SB, SB431542 (an inhibitor of the activin/nodal signalling pathway). Scale bars (b) 100 μm; (h–j) 10 μm; others 25 μm. Figure 2: Retinoid-independent motor neurogenesis from human embryonic stem cells. ( a ) SB431542 treatment from day 0 to 4 followed by puromorphamine from day 4 to 12, with pan-retinoid antagonists from day 4 onwards. ( b ) OLIG2 immunocytochemistry (green) of day 12 hESC-NPCs derived in retinoid-free conditions (−/+ pan-retinoid antagonists). Quantitative OLIG2 immunocytochemistry comparing retinoid-independent culture conditions with ( c ) control conditions and ( d ) retinoid-treated conditions. All cultures were treated with 10 ng ml −1 FGF2 from day 4 to 12. On terminal differentiation ( e ) β-III-TUBULIN (βIII)/SYNAPSIN expression occurs within 4–7 days and ( f ) HB9 expression after 4–5 weeks. ( g ) Quantitative immunocytochemistry for HB9/β-III-TUBULIN co-expressing cells. Co-culture of RA-independent MN precursors with C2C12-derived myotubes for 12 days results in ( h ) outgrowth of neurite tips, ( i ) Tetramethyl Rhodamine Iso-Thiocyanate (TRITC)-α-bungarotoxin plaques on myotubes and ( j ) neuromuscular synapse formation. ( k ) Current-clamp recording from RA-independent MNs (56 days post-plating): injection of positive current generates action potentials that are blocked by voltage-dependent Na + channel blocker tetrodotoxin (TTX; 300 nM). Voltage-clamp recordings from RA-independent MNs, held at −60 mV, showing responses to application of the ionotropic glutamate receptor agonists α-amino-3-hydroxyl-5-methyl-4-isoxazole-propionate (AMPA; 50 μM) and N -methyl- D -aspartic acid (NMDA; 100 μM) and to the inhibitory neurotransmitter, γ-aminobutyric acid (GABA; 50 μM). The lower two traces in this panel show TTX-insensitive miniature excitatory postsynaptic currents (mESPCs), recorded in the presence of picrotoxin (50 μM) and under conditions in which NMDA receptors would be blocked by magnesium ions (Mg 2+ ) present in the external recording solution. Calibration bars for current-clamp recordings, 16 mV and 400 ms; for agonist-evoked whole-cell currents, 80 pA and 4 s; and for mEPSCs, 16 pA and 80 ms. To confirm MN identity, post hoc staining with choline acetyltransferase (ChAT) was conducted. Error bars in c , d and g represent s.e.m, *** P <0.001, Mann–Whitney rank-sum test, a minimum of three biological repeats were performed for each experiment. Ctrl, control; DAPI, 4,6-diamidino-2-phenylindole; mESPCs, miniature excitatory postsynaptic currents; MN, motor neuron; NS, not significant; NPC, neural precursor cell; P, puromorphamine (sonic hedgehog agonist); RA, retinoic acid; SB, SB431542 (an inhibitor of the activin/nodal signalling pathway). Scale bars ( b ) 100 μm; ( h–j ) 10 μm; others 25 μm. Full size image We next investigated the functional maturation of RA-independent MNs. MN precursors co-cultured with C2C12 cell-derived myotubes resulted in putative synaptic connections within 12 days, as demonstrated by the presence of α-bungarotoxin plaques on myotubes (indicating clustering of acetylcholine receptors) contacted by the tips of neurite processes ( Fig. 2h–j ). This is consistent with potential synaptic connectivity of the resulting MNs. Electrophysiological assessment of RA-independent MNs ( Fig. 2k ) showed them to fire tetrodotoxin (TTX)-sensitive action potentials when injected with depolarizing currents. In addition, they possessed receptors for ionotropic glutamate receptors, as evidenced by whole-cell current recordings in response to the application of α-amino-3-hydroxyl-5-methyl-4-isoxazole-propionate (AMPA) and N -methyl- D -aspartic acid (NMDA). Receptors for the inhibitory neurotransmitter, γ-aminobutyric acid, were also present in these cells. Finally, synaptic connectivity was evident by the presence of TTX-insensitive miniature excitatory synaptic postsynaptic currents. Together, these data are consistent with the generation of functional human MNs, independent of retinoid signalling. Retinoid-independent MNs exhibit distinct subtype diversity Although retinoid-independent motor neurogenesis from hESCs has been demonstrated ( Fig. 2 ), we found that exogenous RA increased both the OLIG2-expressing precursor population ( Fig. 2d ; 50.92±2.5% with RA versus 36.5±3.0% in RA-independent culture conditions, P <0.001) and the number of post-mitotic MNs ( Figs 1l and 2g ; 17.5±1.2% versus 11.2±0.9%, P =0.0071). Therefore, we next considered whether retinoid signalling influences the repertoire of specific MN subtypes generated. The diversity and number of MNs required at different levels of the neuraxis are determined by codes of HOX and LHX gene expression [19] , [20] . Although HOX genes are directly regulated by RA, the absolute dependence varies for individual HOX genes; therefore, the HOX gene expression profile would be expected to vary in RA-treated and RA-independent groups. Transcriptional profiling revealed differential HOX gene upregulation in the RA-treated versus RA-independent conditions, suggesting that RA-independent motor neurogenesis occurs with distinct rostrocaudal identities ( Fig. 3a–c ). The relative expression profiles of HOX genes, determined by quantitative RT–PCR (qRT–PCR), showed that RA-independent cultures had significantly reduced expression of anterior HOX genes, including HOXB1 and HOXA3 , compared with the more caudal markers, suggesting a preferential differentiation of caudal rather than rostral MNs. Quantitative immunocytochemistry of MN precursors derived in both RA-independent and RA-treated conditions ( Fig. 3d,e ) reinforced transcriptional studies by demonstrating significantly higher expression of HOXB4 and HOXC9 in retinoid-treated cultures ( Fig. 3e ; 9.6±1.5% versus 4.2±0.7%, P =0.0096; 22.9±1.6% versus 12.4±1.8%, P =0.0002, respectively), while the caudal/lumbar marker HOXC10 was expressed at a significantly higher level in RA-independent conditions ( Fig. 3e ; 6.1±1.2% versus 1.9±0.6%, P =0.0094). To confirm whether this bias was maintained following further neuronal differentiation, we analysed expression of relevant HOXC genes [30] by qRT–PCR and immunocytochemistry in terminally differentiated MNs derived from both RA-independent and RA-treated protocols. This demonstrated a similar bias to the caudal spinal cord in RA-independent conditions ( Fig. 3f–h ). Significantly, the RA-independent cultures generated a greater number of HOXC10 and ChAT co-expressing MNs than the RA-treated cultures ( Fig. 3g,h ; 3.8±0.6% versus 1.5±0.4% of total cells co-expressing HOXC10 and ChAT, P =0.0082), representing ∼ 40% of all MNs in RA-independent conditions, given that 9.7±0.8% of these cultures were MNs ( Supplementary Fig. S2 ). 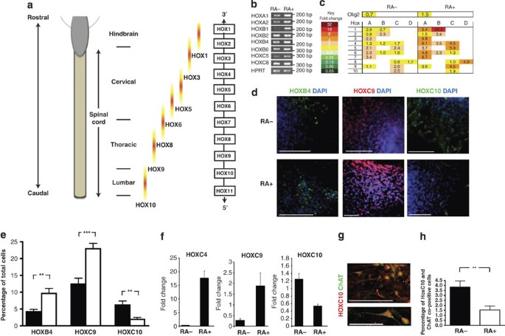Figure 3: Distinct rostro-caudal specification of retinoid-independent motor neurons. (a) A cartoon schematic depicts expression patterns of chromosomally linkedHOXgenes along the R-C axis.HOXgenes at one end of the cluster are expressed more rostrally, whereas those at the opposite end are expressed caudally, as indicated. (b) Reverse transcriptase PCR (RT–PCR) and (c) quantitative RT–PCR (qRT–PCR) of multipleHOXgenes across both experimental conditions (RA-independent and RA-treated), depicted as aHOXgene expression heat map (letters A, B, C and D in the heat map refer to the fourHOXgene clusters located on different chromosomes, while numbers reflect individual genes of each cluster and determine R-C identity, as shown ina). (d) Immunocytochemistry of HOXB4, HOXC9 and HOXC10 in RA-independent and RA-treated conditions. (e) Quantitative analysis of immunocytochemistry ind(black bars are RA-independent cultures, while the white bars represent RA-treated culture conditions). (f) qRT–PCR of HOXC4, HOXC9 and HOXC10 in terminally differentiated cultures (9 weeks after mitogen withdrawal). (g) Immunocytochemistry of HOXC10 (red) and ChAT (green) co-positive motor neurons (low- and high-power magnification, representative images of HOXC10 and ChAT immunolabelled retinoid-independent motor neurons). (h) Quantitative analysis of HOXC10 and ChAT immunocytochemistry shown ing. Error bars ineandhrepresent s.e.m, **P<0.01, ***P<0.001, Mann–Whitney rank-sum test, a minimum of three biological repeats were performed for each experiment. ChAT, choline actetyltransferase; DAPI, 4,6-diamidino-2-phenylindole; hESC, human embryonic stem cell; MN, motor neuron; NSC, neural stem cell; RA, retinoic acid; RA−, retinoid independent; RA+, retinoid treated; SB, SB431542 (an inhibitor of the activin/nodal signalling pathway). All scale bars 50 μm. Figure 3: Distinct rostro-caudal specification of retinoid-independent motor neurons. ( a ) A cartoon schematic depicts expression patterns of chromosomally linked HOX genes along the R-C axis. HOX genes at one end of the cluster are expressed more rostrally, whereas those at the opposite end are expressed caudally, as indicated. ( b ) Reverse transcriptase PCR (RT–PCR) and ( c ) quantitative RT–PCR (qRT–PCR) of multiple HOX genes across both experimental conditions (RA-independent and RA-treated), depicted as a HOX gene expression heat map (letters A, B, C and D in the heat map refer to the four HOX gene clusters located on different chromosomes, while numbers reflect individual genes of each cluster and determine R-C identity, as shown in a ). ( d ) Immunocytochemistry of HOXB4, HOXC9 and HOXC10 in RA-independent and RA-treated conditions. ( e ) Quantitative analysis of immunocytochemistry in d (black bars are RA-independent cultures, while the white bars represent RA-treated culture conditions). ( f ) qRT–PCR of HOXC4, HOXC9 and HOXC10 in terminally differentiated cultures (9 weeks after mitogen withdrawal). ( g ) Immunocytochemistry of HOXC10 (red) and ChAT (green) co-positive motor neurons (low- and high-power magnification, representative images of HOXC10 and ChAT immunolabelled retinoid-independent motor neurons). ( h ) Quantitative analysis of HOXC10 and ChAT immunocytochemistry shown in g . Error bars in e and h represent s.e.m, ** P <0.01, *** P <0.001, Mann–Whitney rank-sum test, a minimum of three biological repeats were performed for each experiment. ChAT, choline actetyltransferase; DAPI, 4,6-diamidino-2-phenylindole; hESC, human embryonic stem cell; MN, motor neuron; NSC, neural stem cell; RA, retinoic acid; RA−, retinoid independent; RA+, retinoid treated; SB, SB431542 (an inhibitor of the activin/nodal signalling pathway). All scale bars 50 μm. Full size image Although OLIG2 and HOX proteins are expressed in RA-independent conditions, the class-I HD protein PAX6 involved in D-V patterning is not induced (1.5±0.4% versus 13.5±1.4% in the RA-treated group, P <0.0001; Supplementary Fig. S3a,b ). A consequence of reduced PAX6 in RA-independent conditions compared to those with RA is an increase in the population expressing NKX2.2 (15.6±1.2% versus 2.1±0.5% in the RA-treated group, P <0.0001; Supplementary Fig. S3a,b ). This is consistent with in vivo studies confirming that restricted subtypes of MNs can still develop in the absence of Pax6, in association with a dorsal expansion of the Nkx2.2 domain [31] . To further examine MN subtype diversification in RA-independent cultures, we undertook qRT–PCR and immunocytochemical analyses, noting that LMC and medial motor column (MMC) pools have distinct transcriptional profiles [19] , [20] ( Fig. 4a ). Specifically, LHX3, LHX1, RALDH2 and FOXP1 expression can be used to phenotype post-mitotic MNs. qRT–PCR analysis of 9 week terminally differentiated MNs showed that RA-independent cultures expressed low levels of RALDH2 and LHX1 in contrast to high expression in RA-treated cultures ( Fig. 4b,c ), suggesting an RA-mediated MN subtype bias to the LMCs. In contrast, LHX3 expression was similar in the two groups ( Fig. 4d ), suggesting that retinoid signalling may be dispensable for specifying medial MMC identity. To corroborate these observations, FOXP1 expression in terminally differentiated mature MNs was studied by quantitative immunocytochemsitry using an established classification system of high, low and off [30] , in conjunction with the pan-MN marker SMI32 [32] ( Fig. 4e,f,h ). RA treatment generated significantly more FOXP1(high) MNs ( Fig. 4f ; 7.1±0.9% versus 1±0.3%, P <0.0001), consistent with an LMC identity. Interestingly, retinoid-independent MNs showed a significantly higher number of FOXP1(off) MNs ( Fig. 4h ; 74.9±2.2% versus 64.9±2.9%, P =0.0107), consistent with MMC identities (medial and/or lateral). When considered together with the similar LHX3 expression between retinoid-independent and retinoid-treated groups, this data, suggests that lateral MMC (also known as the hypaxial motor column or HMC) MNs are preferentially specified in the RA-independent group. To investigate this further, we performed quantitative immunocytochemistry of LHX3 and SMI32 co-expressing MNs and found no significant difference between RA-treated and RA-independent cultures ( Fig. 4g,h ; 60.5±3.2% versus 65.7±2.9%, P =0.2496), confirming that medial MMC identity is not significantly influenced by retinoid signalling. Importantly, there were significantly fewer LHX3 and SMI32 co-positive MNs than FOXP1(off) but SMI32-positive MNs in the retinoid-independent group only ( Fig. 4h ; 65.7±2.9% versus 74.9±2.2%, P =0.02), again suggesting the presence of a FOXP1(off) and LHX3-negative MN population, a molecular phenotype consistent with lateral MMC (or HMC) identity. Indeed, further immunocytochemical studies not only confirmed the presence of FOXP1(off) and LHX3-negative but SMI32-expressing lateral MMC (or HMC)-like MNs but also further demonstrate that this subtype appears to be preferentially specified in RA-independent cultures ( Fig. 4i,j ; 8.0±1.2% versus 3.3±0.76%, P =0.0029). 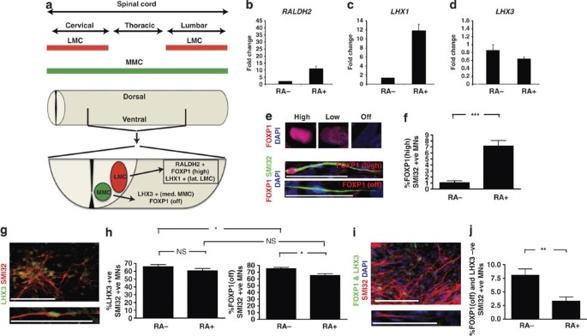Figure 4: Distinct motor columnar identities of retinoid independent motor neurons. (a) A schematic depicts the columnar arrangement and gene expression patterns of specific motor neuron subtypes in relation to different rostro-caudal portions of the neuraxis. QRT–PCR analysis of terminally differentiated MNs (9 weeks after mitogen withdrawal) for lateral motor column (LMC) markers (b) retinaldehyde dehydrogenase 2 (RALDH2) and (c)LHX1.(d) QRT–PCR forLHX3, a marker of the medial division of the medial motor column (MMC). (e) Immunocytochemistry of terminally differentiated MNs for the LMC marker FOXP1. (f) Quantification of FOXP1(high) and SMI32 co-expressing cells. (g) LHX3 and SMI32 immunocytochemistry (low- and high-power magnification, representative images of LHX3 and SMI32 immunolabelled retinoid-independent motor neurons). (h) Quantitative analysis of LHX3 and SMI32 co-expressing cells, and FOXP1(off) and SMI32 co-expressing cells in RA-independent and RA-treated cultures. (i) Immunocytochemistry of FOXP1(off)/LHX3−/SMI32+ cells (low- and high-power magnification, representative images of immunolabelled retinoid-independent motor neurons). (j) Quantified immunocytochemistry of FOXP1(off)/LHX3−/SMI32+ cells. Error bars inf, handjrepresent s.e.m, *P<0.05, **P<0.01, ***P<0.001, Mann–Whitney rank-sum test, a minimum of three biological repeats were performed for each experiment. DAPI, 4,6-diamidino-2-phenylindole; LMC, lateral motor column; MMC, median motor column; NS, not significant; RA, retinoic acid, RA−, retinoid independent, RA+, retinoid treated. All scale bars, 50 μm. Figure 4: Distinct motor columnar identities of retinoid independent motor neurons. ( a ) A schematic depicts the columnar arrangement and gene expression patterns of specific motor neuron subtypes in relation to different rostro-caudal portions of the neuraxis. QRT–PCR analysis of terminally differentiated MNs (9 weeks after mitogen withdrawal) for lateral motor column (LMC) markers ( b ) retinaldehyde dehydrogenase 2 ( RALDH2 ) and ( c ) LHX1. ( d ) QRT–PCR for LHX3 , a marker of the medial division of the medial motor column (MMC). ( e ) Immunocytochemistry of terminally differentiated MNs for the LMC marker FOXP1. ( f ) Quantification of FOXP1(high) and SMI32 co-expressing cells. ( g ) LHX3 and SMI32 immunocytochemistry (low- and high-power magnification, representative images of LHX3 and SMI32 immunolabelled retinoid-independent motor neurons). ( h ) Quantitative analysis of LHX3 and SMI32 co-expressing cells, and FOXP1(off) and SMI32 co-expressing cells in RA-independent and RA-treated cultures. ( i ) Immunocytochemistry of FOXP1(off)/LHX3−/SMI32+ cells (low- and high-power magnification, representative images of immunolabelled retinoid-independent motor neurons). ( j ) Quantified immunocytochemistry of FOXP1(off)/LHX3−/SMI32+ cells. Error bars in f, h and j represent s.e.m, * P <0.05, ** P <0.01, *** P <0.001, Mann–Whitney rank-sum test, a minimum of three biological repeats were performed for each experiment. DAPI, 4,6-diamidino-2-phenylindole; LMC, lateral motor column; MMC, median motor column; NS, not significant; RA, retinoic acid, RA−, retinoid independent, RA+, retinoid treated. All scale bars, 50 μm. Full size image Taken together, the gene expression profiling and immunocytochemical analyses ( Figs 3 and 4 ) provide evidence for a bias in the generation of MN subtype specificity to more caudal (spinal) MMC neurons (comprising both the medial and lateral subdivisions) under RA-independent differentiation conditions. In contrast the output of RA-treated cultures are biased to more rostral populations, with a relative predominance of LMC MNs and medial (but less lateral) MMC identities. These findings suggest a medial MMC ground state, the specification of which appears to be refractory to changes in retinoid signalling. RA exposure then promotes LMC specification at the expense of lateral (but not medial) MMC identity ( Fig. 5 ). 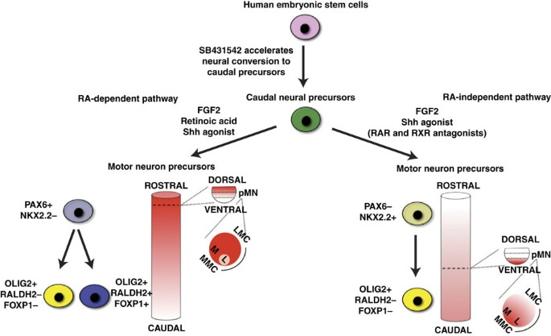Figure 5: Schematic representation of retinoid-dependent and -independent protocols for accelerated motor neurogenesis from hESCs. SB431542 treatment accelerates neural induction and imposes a caudal positional identity. Subsequent treatment with a sonic hedgehog agonist (puromorphamine) and FGF2 (with or without RA) permits the generation of motor neurons. MN derivatives from the retinoid-independent pathway are biased to the caudal spinal cord (as depicted by the distribution and intensity of the red shading), the ventral aspect of the pMN domain and predominantly MMC fates (both medial and lateral subdivisions). MN derivatives from the retinoid-dependent pathway are biased to the rostral spinal cord (as depicted by the distribution and intensity of the red shading), the dorsal aspect of the pMN domain and promote the specification of LMC fates in addition to medial (but not lateral) MMC identities. The medial MMC emerges as a ground state for motor neurogenesis, being seemingly refractory to changes in retinoid signalling. Under retinoid-independent conditions, the lateral division of the MMC is also specified, while RA promotes the specification of LMC identities at the expense of lateral (but not medial) MMC MN specification. FGF2, fibroblast growth factor 2; L, lateral; LMC, lateral motor column; M, medial; MMC, median motor column; RA, retinoic acid; SB431542, an inhibitor of the activin/nodal signalling pathway. Figure 5: Schematic representation of retinoid-dependent and -independent protocols for accelerated motor neurogenesis from hESCs. SB431542 treatment accelerates neural induction and imposes a caudal positional identity. Subsequent treatment with a sonic hedgehog agonist (puromorphamine) and FGF2 (with or without RA) permits the generation of motor neurons. MN derivatives from the retinoid-independent pathway are biased to the caudal spinal cord (as depicted by the distribution and intensity of the red shading), the ventral aspect of the pMN domain and predominantly MMC fates (both medial and lateral subdivisions). MN derivatives from the retinoid-dependent pathway are biased to the rostral spinal cord (as depicted by the distribution and intensity of the red shading), the dorsal aspect of the pMN domain and promote the specification of LMC fates in addition to medial (but not lateral) MMC identities. The medial MMC emerges as a ground state for motor neurogenesis, being seemingly refractory to changes in retinoid signalling. Under retinoid-independent conditions, the lateral division of the MMC is also specified, while RA promotes the specification of LMC identities at the expense of lateral (but not medial) MMC MN specification. FGF2, fibroblast growth factor 2; L, lateral; LMC, lateral motor column; M, medial; MMC, median motor column; RA, retinoic acid; SB431542, an inhibitor of the activin/nodal signalling pathway. Full size image This study demonstrates a novel retinoid-independent pathway for the generation of functional human MNs from ESCs that display a predominantly caudal identity and bias to medial motor columnar pools (both lateral and medial). We and others have previously showed that activin/nodal inhibition with SB431542 accelerates neural conversion from hESCs [25] , [26] , [33] , and this study demonstrates that this system allows accelerated specification of MN progenitors within 12 days compared with most published protocols of ∼ 30 days [1] . Moreover, as neuralization with SB431542 imposes a caudal identity on resulting precursors, we could investigate the necessity of RA for human motor neurogenesis and show that subclasses of MNs can be specified independently of RA in the context of activin/nodal inhibition and hedgehog signalling, thereby increasing the potential diversity of human MNs for study ( Fig. 5 ). This is an important consideration for the creation of accurate disease models of degenerative processes that display selective neuronal subtype vulnerability, as seen in amyotrophic lateral sclerosis and spinal muscular atrophy [3] . Established roles for RA in motor neurogenesis include the upregulation of HOX gene expression [27] ; upregulation of Class I HD genes involved in D-V neural patterning [34] , [35] and the diversification of MN subtypes from post-mitotic MN precursor pools [19] , [20] , [22] . The RA-independent differentiation conditions used here apply sequential extrinsic factors that modulate cell fate, including TGF-β antagonism by SB431542 followed by hedgehog and FGF pathway activation using purmorphamine and FGF2. Under these conditions, ventral fate-determining proteins including NKX2.2 and OLIG2 are expressed. HOX gene expression is increased in response to SB431542 treatment, compared with controls. However the profile of expressed HOX genes varies to that expressed in response to RA [26] . Together, signals that lead to OLIG2 and HOX protein expression, in the absence of RA, provide the essential basis for MN precursor specification in this study. In view of the interplay of FGF and RA signalling in determining caudal identity, it will be of interest to study the specific requirements of FGFs in the context of RA-independent motor neurogenesis [36] , [37] . In vivo , Pax6 functions to establish the pMN domain through cross-repression of the class-II gene Nkx2.2 , limiting its expression to the more ventral p3 domain [5] , [38] . A consequence of reduced PAX6 in RA-independent conditions, compared to those with RA, is an increase in the population expressing NKX2.2. This is consistent with previous studies demonstrating the ability of RA to regulate D-V identity during neural differentiation from mouse embryonic stem cells [39] and additionally with analysis of mutant Pax6 mice, which show a dorsal expansion of the Nkx2.2 domain. Despite the significance of Pax6 in pMN domain development, MNs still develop in Pax6-null rodents, although with reduced numbers and selective loss of specific subgroups of Pax6-dependent MNs [31] , [40] . These in vivo data suggest that, in the absence of RA, the lack of PAX6 in hESC neural derivatives would lead to development of restricted subgroups of MNs. This is the first report demonstrating retinoid-independent specification of functional human MNs. Our findings are consistent with previous observations that have shown that MNs can develop when retinoid signalling is compromised [12] , [41] , and that the necessity for retinoid signalling and its effects on MN output are dependent on developmental context. Retinoid-independent motor neurogenesis occurs in a vitamin-A-deficient quail model system in which embryos display localized disruption of D-V patterning at the cervical but not at more posterior levels of the spinal cord [41] . A differential R-C dependence on RA is consistent with our in vitro findings that show specification of more caudal MN fates in human cells in the absence of RA signalling. In addition, our data suggest that RA-independent motor neurogenesis results in a MMC subtype bias, compatible with the known contribution of RA to subtype diversification [22] . In vivo , FOXP1 is expressed by MNs at brachial, thoracic and lumbar levels of the spinal cord, and its activity mediates translation of the HOX code present in each precursor pool and diverts MNs to LMC fates [30] . Recent evidence suggests a role for HoxC9 as a 'master regulator' of motor system organization through global cross-repressive activities [42] . Interestingly, our data suggests significantly more induction of HOXC9 in retinoid-treated when compared with retinoid-independent cultures (although expression is observed in both conditions; Fig. 3 ). Further manipulation of HOXC9 expression, via extrinsic signals or gene targeting, may facilitate more refined approaches to directed differentiation of hESCs to enriched populations of MN subtypes. Our data demonstrates the emergence of FOXP1(high) (LMC) MNs with continuing retinoid exposure. LMC neurons are only generated at specific HOX levels (brachial and lumbar), which may account for the modest (although significant) increase in the percentage of LMC MNs. Inhibition of retinoid signalling in post-mitotic MNs has been shown to divert their fate, at the expense of LMC, to a lateral MMC (or HMC) identity [19] . The demonstration of an increase in FOXP1(off) MNs on inhibition of retinoid signalling together with no significant difference in LHX3 and SMI32 co-positive cells in both experimental conditions and, more specifically, demonstration of significantly higher numbers of FOXP1(off) and LHX3-negative but SMI32-positive MNs in RA-independent conditions are consistent with these studies. Therefore, retinoid signalling promotes the specification of LMC MNs at the expense of lateral MMC MNs, Furthermore, the refractoriness of the medial MMC to changes in retinoid signalling implicates its development as a MN ground state ( Fig. 5 ). This study supports the view that the retinoid pathway is differentially relevant to distinct stages of motor neurogenesis. The functional implications of these findings are of considerable interest, because motor column organization in development forms the basis for motor pools and target innervation [3] , and in diseases such as amyotrophic lateral sclerosis, MNs have differential vulnerability to degeneration. Thus, it would be of interest to explore behaviour of RA-independent and -dependent MNs in experimental models of injury. Additionally, given a growing interest in the potential use of retinoid pathway manipulation as a neuroregenerative therapy [43] , our study may have implications for either chemical- or cell-based therapeutic strategies for degenerative conditions such as amyotrophic lateral sclerosis and spinal muscular atrophy. Note added in proof: A parallel study using mouse embryonic stem cells has been reported while this work was under consideration (Peljto, M., Dasen, J. S., Mazzoni, E. O., Jessell, T. M. & Wichterle, H. Functional diversity of ESC-derived motor neuron subtypes revealed through intraspinal transplantation. Cell Stem Cell 7 , 355–366 (2010)). hESC culture and neural induction The hESC lines H9 (WiCell Research Institute) and HuES9 (hES facility, Harvard University) were propagated in defined medium supplemented with 8 ng ml −1 of FGF2, 10 ng ml −1 of activin [44] and 10 ng ml −1 of insulin as an adherent culture system on a layer of irradiated mouse embryonic fibroblasts [26] , [45] . Human ESCs were enzymatically passaged in a 1:4 split ratio at the point of subconfluence. To generate neural precursor cells (NPCs), hESCs were enzymatically dissociated, mechanically triturated, centrifuged and washed in fresh medium. Cell aggregates were next suspended in chemically defined medium in 10-cm culture dishes on an orbital shaker. Chemically defined medium consisted of 50% Iscove's modified Dulbecco's medium (IMDM; Gibco) plus 50% F12 plus Glutamax (Gibco), supplemented with 1.75 mM human recombinant insulin (Roche), 0.38mM transferrin (Roche), 450 μM of monothioglycerol (Sigma), 10 μl ml −1 lipids (Sigma) and 5 mg ml −1 bovine serum albumin fraction V (Sigma). SB431542 (10 μM; Tocris Bioscience) was added from day 0–4. Eight-day patterning protocols were developed in which hESC-NPCs were cultured in combinations of FGF2 (10ng ml −1 )/SB431542 (10 μM)/RA (0.1 μM)/puromorphamine [46] (1 μM) for spinal MN specification. For terminal differentiation, hESC-NPCs were plated onto poly( D -lysine)/laminin-coated coverslips and cultured in Dulbecco's modified Eagle's medium (DMEM)/2% B27/1% penicillin/streptomycin/fungizone (PSF), 10 ng ml −1 BDNF (brain-derived neurotrophic factor; R&D Systems) and 10 ng ml −1 GDNF (Glial cell-derived neurotrophic factor; R&D Systems) in the absence of mitogens. The synthesis of retinoid antagonists The synthesis of UVI3003 has been described elsewhere [29] . The synthesis of UVI2024, also called BMS493, follows the methodology described recently for the preparation of the halogenated derivatives [28] . A description of the synthetic method and the characterization data is described in the Supplementary Methods . Reverse transcription PCR Total RNA was extracted from dissociated and washed cells using the RNeasy Mini Kit (Qiagen) following the manufacturer's instructions. cDNA was synthesized from 2 μg of RNA using Moloney murine leukaemia virus reverse transcriptase (Invitrogen) and oligo-dT primers. PCR was carried out using Taq polymerase (Invitrogen). PCR products were separated on a 2% agarose gel and visualized with SYBR-Green (Invitrogen). Primer information is provided in Supplementary Table S1 . Quantitative reverse transcription PCR qPCR was carried out using the DyNAmo HS SYBR-Green qPCR kit (Finnzymes) and an Opticon2 real-time PCR system with Opticon Monitor version 3 software (Bio-Rad Laboratories). Selection of Hprt1 as an appropriate reference gene for these sample sets was carried out, as previously described [47] . Further, during optimization of each gene of interest primer pair, the reaction efficiencies were determined (taking values between 95% and 105% as satisfactory), with product integrity checked using both melting curve and agarose gel analysis. Primer information is provided in Supplementary Table S2 . The data from sample and technical replicates is expressed as fold change (mean±s.e.m. ), determined using the ΔΔCq method with respect to the reference gene. Immunocytochemistry Cells plated down on poly- D -lysine/laminin-coated glass coverslips were fixed with 4% fresh paraformaldehyde for 20 min at room temperature and washed three times with PBS. Samples were next blocked for 1 h with 0.3% Triton/PBS/5% goat serum and then incubated overnight with primary antibody in 0.2% Triton/PBS/2% goat serum at 4°C. After three washes in PBS, secondary antibody (goat anti-mouse, Alexa Fluor 488 or 555, 1:1,000) in PBS/Hoechst (1:4,000) was next applied for 1 h. Primary antibodies included NESTIN (1:500; Chemicon), glial fibrillary acidic protein (GFAP, 1:200; DakoCytomation), OLIG2 (1:200, Chemicon), β-III-TUBULIN (1:500; Sigma-Aldrich), SYNAPSIN (1:500; Calbiochem), NKX6.1 (F65A2), NKX2.2 (74.5A5), PAX6, LHX3 (67.4E12), HOXB4, HOXC10, HB9 (815C10) (all in the ratio 1:50; Developmental Studies Hybridoma Bank), choline acetyltransferase (ChAT, 1:200; Chemicon), SMI32 (1:1,000, Covance), HOXC9 (1:200, Abcam), HOXC10 (1:200, Sigma), LHX3 (1:200, Abcam). Electrophysiological recordings Whole-cell current-clamp and voltage-clamp recordings were made from neurons at room temperature (21±2 °C) using an Axopatch-1C amplifier (Molecular Devices) using methods as described previously [48] , [49] . Briefly, coverslips were transferred to a recording chamber perfused with an external recording solution composed of (in mM) 152 NaCl, 2.8 KCl, 10 HEPES, 2 CaCl 2 , 10 glucose (pH 7.3; 320–330 mOsm). Patch pipettes were filled with a K-gluconate-based internal solution containing (in mM): 155 K-gluconate, 2 MgCl 2 , 10 Na-HEPES, 10 Na-PiCreatine, 2 Mg 2 -ATP and 0.3 Na 3 -GTP (pH 7.3; 300 mOsm). For current-clamp recordings, the external recording solution was supplemented with antagonists of glutamate and γ-aminobutyric acid ligand-gated ion channels (CNQX 5 μM; D-AP5 50 μM; picrotoxin 50 μM; and strychnine 20 μM). For the recording of whole-cell AMPA- and NMDA-evoked currents and synaptically mediated glutamate receptor responses, the external solution was supplemented with picrotoxin (50 μM) and strychnine (20 μM). In all experiments in which NMDA receptor-mediated responses were studied, a saturating concentration of the co-agonist, glycine (50 μM), was also added to the external recording solution. Miniature excitatory postsynaptic currents were recorded in solutions supplemented with 300 nM TTX, picrotoxin (50 μM), strychnine (20 μM) and MgCl 2 (1 mM). Events were recorded for 5–10 min at a holding potential of −70 mV. Nerve and muscle co-culture methods Mouse muscle cell lines (C2C12 myoblasts, ATCC) were cultured with DMEM containing 4.5 g l −1 glucose, 4 mM L -glutamine and 1mM sodium pyruvate, supplemented with 10% fetal bovine serum (Invitrogen) on glass coverslips. Horse serum (10%; Invitrogen) was used to induce myotube differentiation, confirmed using phase-contrast microscopy. Cultures were maintained for 3–7 days before the addition of RA-independent MN progenitors in DMEM/2% B27/1%PSF, 10 ng ml −1 BDNF (R&D Systems) and 10 ng ml −1 GDNF (R&D Systems). Cells were then fixed in 1× PBS containing 4% paraformaldehyde after 7–12 days. Fixed cells were incubated in Tetramethyl Rhodamine Iso-Thiocyanate (TRITC)-α-bungarotoxin (5 μg ml −1 ; Molecular Probes) for 15 min to label acetylcholine receptors on myotubes, TOPRO3 (10 μl ml −1 ; Molecular Probes) for 10 min to label cell nuclei, and primary antibodies against either 150 kDa neurofilament proteins (1:200; Chemicon) or neuronal-specific βIII-tubulin (1:200; Abcam) overnight at 4 °C. Coverslips were then washed in 1× PBS before labelling with swine anti-rabbit FITC-conjugated secondary antibodies (1:40; Dako). Preparations were viewed on a Zeiss LSM510 confocal microscope (Zeiss). Quantification and statistical analysis All analysis was carried out on a minimum of three biological replicates unless otherwise stated. Cell counts were performed across a minimum of five fields of view (approximately 100–300 cells per field) from a minimum of three biological replicates across two different hESC lines. A P -value of <0.05 was considered statistically significant. Values are expressed as the mean±s.e.m. The Mann–Whitney rank-sum test was used for non-parametric analysis using GraphPad Prism 4 (Graph-Pad Software). How to cite this article: Patani, R. et al . Retinoid-independent motor neurogenesis from human embryonic stem cells reveals a medial columnar ground state. Nat. Commun. 2:214 doi: 10.1038/ncomms1216 (2011).